Dynamic optimization identifies optimal programmes for pathway regulation in prokaryotes To survive in fluctuating environmental conditions, microorganisms must be able to quickly react to environmental challenges by upregulating the expression of genes encoding metabolic pathways. Here we show that protein abundance and protein synthesis capacity are key factors that determine the optimal strategy for the activation of a metabolic pathway. If protein abundance relative to protein synthesis capacity increases, the strategies shift from the simultaneous activation of all enzymes to the sequential activation of groups of enzymes and finally to a sequential activation of individual enzymes along the pathway. In the case of pathways with large differences in protein abundance, even more complex pathway activation strategies with a delayed activation of low abundance enzymes and an accelerated activation of high abundance enzymes are optimal. We confirm the existence of these pathway activation strategies as well as their dependence on our proposed constraints for a large number of metabolic pathways in several hundred prokaryotes. The consideration of organisms based on optimality principles has provided explanations for a large number of important biological phenomena [1] , [2] , [3] , [4] , [5] , [6] . An important component of the adaptation of organisms is the ability to quickly adapt to changes in their natural environment to survive and prevail against competitors [6] , [7] , [8] , [9] , [10] . With only a limited amount of resources available, the ability of a quick adaptation can provide an important evolutionary advantage. In this work, we study optimal programmes for the activation of metabolic pathways under the constraint of a limited cellular protein synthesis capacity. Being able to quickly adjust fluxes through metabolic pathways is of critical importance to reduce lag times upon depletion of essential biomass components and during major growth transitions [6] , [7] , [11] , [12] . Previous work has established that, assuming a limited total abundance of proteins as well as the minimization of the invested protein, a sequential induction of enzymes along a pathway is optimal for a rapid activation [13] , [14] , [15] , [16] , [17] , [18] , [19] . That metabolic pathways show a pattern of sequential activation, also known as just-in-time-activation [19] , has been demonstrated experimentally in Escherichia coli for a selected number of amino-acid biosynthetic pathways [18] and on a global scale in Saccharomyces cerevisiae [20] . However, previous works trying to explain these patterns face several problems. First, they predict that a sequential activation of enzymes within a linear metabolic pathway is always preferential to other types of activation strategies. This result is problematic in that the partial operonic organization of many metabolic pathways in prokaryotes prohibits a detailed sequential activation of proteins within a pathway, as proteins on a monocistronic transcript are produced with only a small delay [21] , [22] . To some extent, these observations can be explained by a balance between the fitness advantage obtained through a sequential activation of enzymes within a pathway and the fitness advantage of an operonic organization that minimizes biochemical noise [23] , [24] and reduces the length of promoter sequences [18] . Second, although the production of proteins represents a burden for the cell [25] , [26] , previous approaches only incompletely took into account that protein cost lies in the process of their production ( cf . ref. 26 ) or even assumed that proteins can be produced at any rate [13] , [14] , [15] , [16] , [19] . Here we use dynamic optimization to investigate how limitations in protein production capacity influence the optimal timing of the production of enzymes to activate a metabolic pathway. We find that the interplay between the protein production capacity of the cell and the amount in which a particular enzyme needs to be produced (that is, its abundance) can explain the optimality of a wide variety of pathway activation strategies. In particular, we find that the previously reported sequential activation strategy of enzymes along a pathway [13] , [14] , [15] , [16] , [17] , [18] , [19] is only optimal if large amounts of proteins need to be produced, whereas the simultaneous activation of all enzymes within a pathway is optimal in the case where only small amounts of protein need to be produced. Thus, we show that, depending on protein abundances, an operonic organization of a metabolic pathway is optimal to reduce activation time, whereas previous work postulated activation time-independent effects to explain the operonic organization of metabolic pathways [18] , [23] . Moreover, we observe that, if there are differences in the abundance of enzymes of a pathway, it is optimal to produce enzymes with high abundance earlier and to delay the production of enzymes with low abundances. Enzyme synthesis capacities influence activation strategies We consider the activation of a metabolic pathway that comprises four enzymatic steps e 1 , …, e 4 that convert a buffered substrate S via three intermediates Y 1 , …, Y 3 into a product P ( Fig. 1a , Methods). In many cases, the activation of a particular pathway is required to resume growth, for instance, if an amino acid that has been depleted from the growth medium has to be synthesized. If a particular pathway product p ( t ) has a fixed proportion in cellular biomass, growth cannot resume unless the pathway product is present in sufficient quantities. An example for a mechanism implementing such a pathway-dependent growth control is the stringent response in E. coli that arrests growth if there is a lack of amino acids [27] . 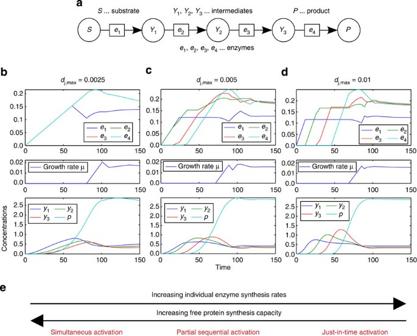Figure 1: Model pathway and optimal activation strategies. (a) Illustrates the metabolic pathway under study. The individual enzyme synthesis rates aredj,max=0.0025 inb,dj,max=0.005 inc,dj,max=0.01 indand the free protein synthesis capacity is set todmax=0.01. For each case, the optimal enzyme profiles, growth rate and the corresponding metabolite profiles are shown. This and all other figures present the concentration profiles and simulation time in arbitrary units. Ine, the influence of enzyme synthesis rate relative to the free protein synthesis capacity on optimal activation strategies is summarized. Therefore, we introduce an objective function that maximizes biomass formation limited by the synthesis of the product of the considered pathway Figure 1: Model pathway and optimal activation strategies. ( a ) Illustrates the metabolic pathway under study. The individual enzyme synthesis rates are d j, max =0.0025 in b , d j, max =0.005 in c , d j, max =0.01 in d and the free protein synthesis capacity is set to d max =0.01. For each case, the optimal enzyme profiles, growth rate and the corresponding metabolite profiles are shown. This and all other figures present the concentration profiles and simulation time in arbitrary units. In e , the influence of enzyme synthesis rate relative to the free protein synthesis capacity on optimal activation strategies is summarized. Full size image where μ is the growth rate. Here the time courses of the enzymes e 1 ( t ), …, e 4 ( t ) and growth rate profile μ ( t ) are determined to maximize the objective function. As we consider the activation of the pathway to an active state, which is maintained after activation, a large final time t f is defined (assumed to be t f =1,000 arbitrary time units). By explicitly taking into account the growth rate in the course of pathway activation, we are able to more precisely model the influence of dilution through growth on pathway activation. The concentration of an enzyme e j ( t ) is determined by two factors: the enzyme synthesis rate d j ( t ) and the dilution through growth μ ( t )· e j ( t ). We assume that dilution through growth is the major source for protein degradation as it has been reported previously for E. coli [28] . There are two constraints on enzyme synthesis rate: the synthesis capacity of individual enzymes and the free protein synthesis capacity of the cell. For each enzyme, there is an upper bound on the rate at which it can be synthesized, d j, max . This upper bound is determined by several factors such as the maximal copy-number of the associated messenger RNA and its translation efficiency [29] . Depending on the required concentration of an enzyme for an active pathway (that is, its abundance), both factors can be adjusted in the course of evolution to increase and decrease the production capacity of the enzyme. In consequence, enzyme abundance is a major determinant in the maximal production capacity of an enzyme. Thus, the time course of e j is determined by The free protein synthesis capacity corresponds to the maximal amount of protein that can be produced by free ribosomes of the cell within a specific time interval. We use the constraint based on free-protein synthesis capacity to account for the synthesis of other proteins by ribosomes that need to be produced to maintain cell viability [30] . The free protein synthesis capacity is mainly determined by ribosomal concentrations, total mRNA concentrations, transfer RNA concentrations and the availability of substrates for protein synthesis. Thus, we formulate the constraint on free-protein synthesis capacity, d max , within a specific time interval by In the first step, we analysed the influence of the interplay between individual enzyme synthesis and free protein synthesis capacity on optimal pathway activation strategies for a prototypic metabolic pathway with unit kinetic parameters ( Fig. 1a ). If the sum of individual enzyme synthesis rates is equal (or smaller) than the free protein synthesis capacity, all enzymes can be produced at the same time and, hence, they are induced simultaneously for a rapid pathway activation ( Fig. 1b ). To give a clear illustration, we reduced the plotted time window to the dynamics of the pathway activation (the complete profiles are shown in Supplementary Fig. S1 ). In Fig. 1d , we consider the case where each individual enzyme synthesis rate is equal to the free protein synthesis capacity. This corresponds to enzymes that have to be produced in large amounts. For this scenario, we observe a sequential activation of enzymes according to their order within the pathway. This type of activation strategy is similar to the so called ‘just-in-time-activation’ strategy [19] , also reported in other studies [13] , [14] , [15] , [16] . In the case in which each individual enzyme synthesis rate is smaller than the free protein synthesis capacity but their sum is larger than the free protein synthesis capacity, we observe an intermediary behaviour in which parts of the metabolic pathway are sequentially activated ( Fig. 1c ). The influences of the different constraints on optimal pathway activation strategies are summarized in Fig. 1e . To investigate the influence of kinetic parameters on the optimization runs in the previous section, we repeated the optimization for 100 uniformly sampled kinetic parameter sets from the interval [0,2] for several values of the individual enzyme synthesis capacity. Although a sequential or partial sequential activation of enzymes within the model pathway is often optimal, we observed many cases in which the order of activation is rearranged such that the production of later steps of the pathway is induced before the induction of earlier steps. A closer investigation showed that the rearrangement of the activation sequence from the order of reactions in the pathway is because of differences in the abundance of individual enzymes caused by differences in their catalytic efficiency. We observed that enzymes that need to be present in higher amounts relative to the other enzymes of the pathway are induced earlier than enzymes with average abundances as their production takes longer ( Fig. 2 ). Moreover, we observed that enzymes whose abundance is low relative to the other enzymes of the pathway tended to be activated later than surrounding enzymes of the pathway ( Fig. 2 ). For similar plots for all considered individual enzyme synthesis rates see Supplementary Fig. S2 . 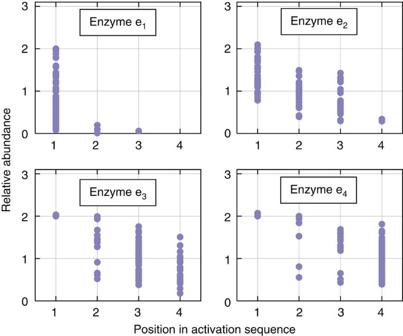Figure 2: Influence of enzyme abundance on the order of activation of enzymes in a pathway. Position of each enzyme in the activation sequence for 100 randomly drawn kinetic parameter sets for an individual enzyme synthesis rate ofdj,max=0.005. Thexaxis denotes the position in the activation sequence defined as the rank of the activation time of the particular enzyme in the ordered list of activation times for this parameter set. Theyaxis indicates the abundance of each enzyme relative to the average abundance of enzymes for each particular set of kinetic parameters. Whereas the production of high abundance enzymes is induced earlier, low abundance enzymes tend to be activated later than the surrounding enzymes of the pathway. Figure 2: Influence of enzyme abundance on the order of activation of enzymes in a pathway. Position of each enzyme in the activation sequence for 100 randomly drawn kinetic parameter sets for an individual enzyme synthesis rate of d j, max =0.005. The x axis denotes the position in the activation sequence defined as the rank of the activation time of the particular enzyme in the ordered list of activation times for this parameter set. The y axis indicates the abundance of each enzyme relative to the average abundance of enzymes for each particular set of kinetic parameters. Whereas the production of high abundance enzymes is induced earlier, low abundance enzymes tend to be activated later than the surrounding enzymes of the pathway. Full size image Influence of activation strategies on operonic organization To validate the prediction of the optimality of different type of activation strategies depending on enzyme synthesis constraints, we used the operonic organization of enzymes belonging to the same metabolic pathway. Please note that we use the term ‘operon’ synonymously for ‘transcription unit’ for the sake of clarity although, strictly speaking, an operon needs to be composed of at least two genes. An important feature of operons is that the genes contained within them are expressed almost simultaneously [21] , [22] . Thus, in contrast to a regulon, where several genes are controlled by the same transcription factor, and can be activated at the same time or in a sequential fashion, the operonic organization of genes always leads to their almost simultaneous activation. An important conclusion of our predictions is that the number of genes that are activated simultaneously should decrease with increasing enzyme synthesis rates relative to the free-protein synthesis capacity. To test this hypothesis in our optimization runs, we assumed that genes that are activated within a certain time span belong to the same operon (Methods) and determined the average number of genes per operon (GpO) for different values of the individual enzyme synthesis rates. Plotting the average number of GpO over different individual enzyme synthesis rates, we observed a decreasing size of operons with increasing individual enzyme synthesis rates ( Fig. 3a ). Thus, when individual enzyme synthesis rates are increasing relative to free protein synthesis capacity, the size of operons decreases. 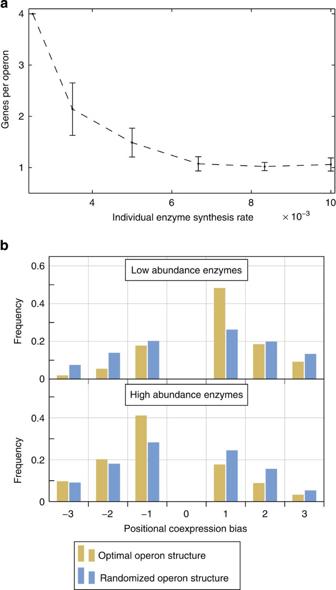Figure 3: Signatures of pathway activation strategies from optimization runs. (a) Influence of individual enzyme synthesis rates on operon size. Enzymes were grouped into operons if the period between the activation time of two enzymes was below a threshold value. Average number of GpO for 100 optimization runs with randomized kinetic parameters has been determined for different individual enzyme synthesis rates (error bars indicate s.d.). (b) Distribution of positional coexpression bias values for low abundance and high abundance enzymes. Frequencies of occurrences of positional coexpression bias values for the optimized (orange) and the randomized operonic organization (blue) from optimization runs with randomized kinetic parameters. Figure 3: Signatures of pathway activation strategies from optimization runs. ( a ) Influence of individual enzyme synthesis rates on operon size. Enzymes were grouped into operons if the period between the activation time of two enzymes was below a threshold value. Average number of GpO for 100 optimization runs with randomized kinetic parameters has been determined for different individual enzyme synthesis rates (error bars indicate s.d.). ( b ) Distribution of positional coexpression bias values for low abundance and high abundance enzymes. Frequencies of occurrences of positional coexpression bias values for the optimized (orange) and the randomized operonic organization (blue) from optimization runs with randomized kinetic parameters. Full size image Another important aspect of our optimization is that, depending on their abundance relative to the remaining enzymes of the pathway, enzymes should be earlier or later activated. Translated into the terms of genes that are coexpressed together in operons, we would expect that genes that have higher abundances relative to other enzymes of a pathway tend to be coexpressed with earlier enzymes of the same pathway, whereas enzymes with lower abundance should be coexpressed with later enzymes of the pathway. To test whether we could find this relationship in our optimization runs, we determined the distribution of the positional coexpression bias values of low abundance and high abundance enzymes across our optimization experiments ( Fig. 3b ). This distribution indicates how often a specific set of enzymes is coexpressed (that is, within the same operon) with earlier or later enzymes of the same pathway (Methods). We compared the distribution of the positional coexpression bias with the optimized operon structure to the distribution we obtained for a random assignment of genes to operons. We found that low abundance enzymes are significantly more often coexpressed with later enzymes of a pathway (Wilcoxon test P -value=6.61 × 10 −4 ), whereas high abundance proteins are significantly more often coexpressed with earlier enzymes of a pathway (Wilcoxon test P -value=3.38 × 10 −7 ). Genomic signatures of activation strategies To test whether the interplay between enzyme synthesis rates and free-protein synthesis capacity has the predicted influence on pathway activation strategies, we analysed the operonic organization of metabolic pathways across all the pathways contained in 550 prokaryotes of the MicroCyc collection [31] , for which information on the operonic structure from MicrobesOnline is available [32] . We tested two types of predictions. First, we investigated the influence of enzyme synthesis rates and free protein synthesis capacity on the size of the operons of specific metabolic pathways. Second, we analysed the influence of protein abundance on the order in which proteins within a pathway are activated. To exclude the possibility that there is a general trend for operon sizes to decrease with increasing protein abundance that is unspecific for metabolic pathways, we determined the correlation between protein abundance and operon size for each of the 550 organisms from MicroCyc. We found that in the vast majority of organisms, operon sizes increase with protein abundances, which is opposite to our predictions ( Supplementary Note 1 ). As measurements on enzyme synthesis rates/protein abundance and free protein synthesis capacity are not available across all of the organisms that we consider, we used genomic features that have a strong influence on these variables for each organism. There are two important factors influencing the free protein synthesis capacity of a cell. The first is the concentration of ribosomes in the cell and the second is the number of protein-coding genes in the genome of an organism. As a reference for the protein synthesis capacity of an organism, we used the copy-number of the ribosomal RNAs in its genome. A correlation analysis across several species shows that there is a strong correlation between both factors (see Supplementary Note 2 ). Another factor that has a strong influence on the free protein synthesis capacity of an organism is the number of protein-coding genes contained within its genome. If the enzymes of a pathway need to be expressed, only a small fraction of the entire cellular protein synthesis capacity will be allocated to the production of these proteins, as proteins required for other functions of the cell need to be produced at the same time [30] . Hence, if considering all other factors such as total ribosomal capacity as equal, an increasing number of protein-coding genes within a genome will reduce the free protein synthesis capacity that can be reallocated to the production of the enzymes of a pathway. This is confirmed by a strong positive correlation between the number of protein-coding genes and the copy-number of ribosomal RNAs across 130 species (see Supplementary Note 2 ). One genomic feature that is often used as a proxy for protein abundance is the codon adaptation index that is computed from the coding sequence of a gene [33] . This measure determines the expression strength of a protein by comparing its codon usage with the codon usage in high-expressed genes [33] such as ribosomal genes. In Supplementary Notes 3 and 4 , we show that codon adaptation indices are a good proxy for protein abundance and are comparable across species. Enzyme synthesis capacities influence operon sizes Following the prediction of our optimization results, we expect that the number of protein-coding genes, the number of rRNA operons as well as enzyme abundance have an influence on the size of metabolic operons. First, we expect the size of the operons, across which the genes of a pathway are distributed, to decrease with an increasing number of protein-coding genes because of a concomitant decrease in the free protein synthesis capacity (hypothesis 1). Second, we expect the size of the operons of a pathway to increase with an increasing number of rRNA operons because of an increase in the free protein synthesis capacity (hypothesis 2). Third, we expect the size of the operons of a pathway to decrease with an increase in the average abundance of enzymes within this pathway (hypothesis 3). We tested these hypotheses across the metabolic pathways of 550 prokaryotes contained in MicroCyc [31] . We analysed only metabolic pathways that are present in at least 100 organisms (99 metabolic pathways). To analyse the above hypotheses, we determined for each organism and each pathway the number of operons across which this pathway is distributed. Then we computed the Spearman’s correlation between the factors outlined in the hypotheses while controlling for the other investigated factors. Moreover, to exclude effects outside metabolism that have an effect on operon sizes, we also controlled for the average size of non-metabolic operons for each organism. For more information about how we controlled for confounding influences on operon sizes, see the Methods section and Supplementary Note 5 . Subsequently, we corrected all of the resulting P -values for multiple testing using the Benjamini–Yekutieli procedure [34] , and only accepted correlations as significant if they were below a false discovery rate of 5%. For 69 of the 99 pathways, we found at least one significant correlation for one of the tested hypotheses ( Table 1 ). For detailed information including P -values across all 99 tested pathways, see Supplementary Data 1–7 . Overall, hypothesis 1 is confirmed for 22 of the 99 pathways and rejected (that is, significant correlation in the opposite direction) for 4 pathways. Hypothesis 2 is confirmed for 29 pathways and rejected for 9 pathways. Hypothesis 3 is confirmed for 32 pathways and rejected for 8 pathways. Of the 69 metabolic pathways with at least one significant correlation, 20 fulfill at least two of the hypotheses and 5 fulfill all of the hypotheses ( Table 1 ). We found only two pathways for which two of the hypotheses are rejected. Among the pathways that fulfilled at least two hypotheses, we found 6 pathways associated to amino acid biosynthesis (among 15 such pathways in the 99 pathways), 3 pathways associated to nucleotide biosynthesis and several pathways associated to producing cofactors. Of the five pathways for which all three hypotheses are confirmed, three belong to amino-acid biosynthetic pathways (leucine, proline and tryptophan biosynthesis). Table 1 Validation of pathway activation strategies Full size table These results show that, although not all hypotheses are confirmed at the same time for many pathways, individual enzyme synthesis rates and free protein synthesis capacity have a strong influence on the size of metabolic operons. This is apparent from the much larger number of 83 confirmations of our hypotheses in comparison with only 21 rejections across all pathways. Moreover, our analysis focuses on pathways whose products are essential for growth. Not all biomass components can be considered equally important for growth and the evolutionary pressure to implement the activation programmes that we propose is expected to be higher for products that are of central importance during most growth transitions. This is exemplified by amino acid biosynthetic pathways, whose activation is essential for a resumption of growth under most conditions. Among the 99 pathways that we considered in our analysis, 15 belong to amino-acid biosynthesis. Considering the 20 pathways for which at least two hypotheses were fulfilled, 6 correspond to amino-acid biosynthetic pathways, which is a significant enrichment (hypergeometric test P -value=1.1 × 10 −2 ). Protein abundance influences the timing of activation A second important prediction of our optimization approach is that the abundance of an enzyme relative to the remaining enzymes of a pathway should have an influence on the order of activation of these enzymes. Reanalyzing the data of previous works on the timing of the activation of enzymes in the arginine biosynthetic pathway of E. coli [19] confirms this result: ArgG, which is the most abundant enzyme of arginine biosynthesis [6] , is activated much earlier than the surrounding steps of the pathway ( Supplementary Note 7 and Supplementary Fig. S3 ). In their work, Zaslaver et al . [19] argued that this discrepancy might be because of pathway topology as ArgG condenses the products of two branches of the arginine biosynthetic pathway. However, we show that our findings also apply to linear chains of reactions that are embedded into more complex pathway topologies ( Supplementary Fig. S3 ). If protein abundance has the predicted influence on the order of activation of enzymes within a pathway, we would expect that abundant enzymes tend to be expressed together with earlier steps of the same pathway, whereas less abundant enzymes are more often coexpressed with later steps of the same pathway. To test this relationship, we computed the average coexpression bias of high and low abundance enzymes across all organisms of the MicroCyc collection. As described above, the average coexpression bias of an organism for high and low abundance enzymes indicates how often a specific set of enzymes is coexpressed with earlier or later steps of a pathway. To exclude effects that result from dependencies between pathway position and protein abundance, we compared, for each organism, the average coexpression bias that can be obtained for the actual operon structure with the average coexpression bias of a randomized operonic organization (see Methods). The actual operonic organization leads to a significantly later activation of low abundance enzymes compared with the randomized operon structure (Wilcoxon test P -value=1.1 × 10 −8 , Fig. 4 ). The average positional coexpression bias for each organism can be found in Supplementary Data 3 . For high abundance enzymes, we find that they are activated significantly earlier through the actual operonic structure in comparison with a randomized operonic structure (Wilcoxon test P -value=2.1 × 10 −4 , Fig. 4 ). Thus, as predicted by the optimization, the operonic structure of metabolic pathways is tuned to a later activation of low abundance enzymes, whereas high abundance enzymes tend to be activated earlier. 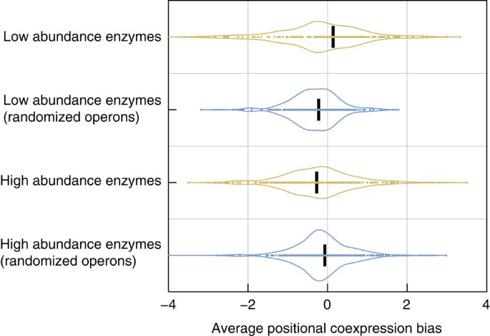Figure 4: Protein abundance has an influence on the timing of pathway activationin vivo. We determined the average positional coexpression bias for each organism of the MicroCyc collection31for low and high abundance enzymes, given the actual operon structure (orange values) and a randomized operon structure (blue values). Each point corresponds to the average positional coexpression bias of an organism. Lines indicate the distribution of these values. Black bars denote the median of each distribution. Only data for organisms that had at least one low abundance enzyme or high abundance enzyme coexpressed with at least one other enzyme in an operon in the pathway shown (293 and 327 organisms, respectively). Figure 4: Protein abundance has an influence on the timing of pathway activation in vivo . We determined the average positional coexpression bias for each organism of the MicroCyc collection [31] for low and high abundance enzymes, given the actual operon structure (orange values) and a randomized operon structure (blue values). Each point corresponds to the average positional coexpression bias of an organism. Lines indicate the distribution of these values. Black bars denote the median of each distribution. Only data for organisms that had at least one low abundance enzyme or high abundance enzyme coexpressed with at least one other enzyme in an operon in the pathway shown (293 and 327 organisms, respectively). Full size image In this work, we used dynamic optimization for the identification and validation of optimal regulatory strategies for controlling metabolic pathways across a large number of metabolic pathways in several hundred prokaryotes. We based our investigation on the assumption of limitations in individual and free protein biosynthesis capacities [26] . The results of the dynamic optimization and the validation show that protein abundance is an important factor influencing the type of regulatory programme that is used to control metabolic pathways. Whereas a low abundance of proteins leads to the optimality of a simultaneous activation of all enzymes of a pathway, a sequential activation of enzymes is optimal in case of high abundance proteins. Depending on the relative abundances of enzymes within a pathway, particularly abundant enzymes are activated much earlier than the preceding reaction steps, whereas enzymes with low abundance tend to be activated later than the neighbouring steps of the pathway. Thus, in contrast to the results of previous works, we show that the sequential activation of enzymes along a pathway, known as ‘just-in-time activation’, is only a special case for quick pathway activation. Another important conclusion that can be drawn from our results is that, depending on environmental conditions, there can be a shift in the optimal programme to activate a pathway. As ribosomal capacity correlates with growth rate, it is optimal to simultaneously activate the enzymes within a pathway in a condition supporting high growth rates while it could be optimal to sequentially activate enzymes in a condition only supporting low growth rates. This observation can explain why the sequential activation of the arginine biosynthetic pathway reported in E. coli [19] was not observed in conditions supporting higher growth rates in a recent work [35] . As an important factor that is representative of the specific type of regulatory programme that is used to control a metabolic pathway, we identified the operonic organization of enzymes within a pathway. The correlations between genomic features as well as operon sizes for different metabolic pathways that we determined show that operon sizes decrease with increasing protein abundance and increase with increasing protein synthesis capacity. Thus, the interplay between protein abundance and constraints in protein synthesis capacity also represents an important driving force in the growth and decline of metabolic operons. As the optimal abundance of proteins as well as the protein synthesis capacity of an organism change in the course of its evolutionary history, the optimal operonic organization of metabolic pathways constantly changes. Thus, protein abundance as well as protein synthesis capacity are important contributors to the often observed high evolutionary plasticity of operons [36] , [37] . We expect that our results are of high importance also beyond the level of metabolism, for instance, for the production of complex molecular machineries such as flagella [38] or in stress responses [39] that require the production of large amounts of protein. Moreover, our results are of relevance for biotechnological applications as they provide guidelines about how a production process should be initiated on the enzymatic level to maximize yield of the product while minimizing the burden on the target organism. Optimal regulatory strategies of metabolic pathways In this work, we consider the activation of a metabolic pathway with a buffered substrate shown in Fig. 1a . Taking into account the dilution of intermediates by growth rate μ ( t ), we obtain: and The kinetic behaviour of metabolites is modelled by irreversible Michaelis–Menten kinetics with the buffered substrate s= 1 (arbitrary concentration unit), for example, (here i= 4). The kinetic parameters are set to or randomly chosen. The initial concentrations are x 1 (0) =x 2 (0) =x 3 (0) =x 4 (0)=0 (arbitrary concentration units) by assuming a complete inactive pathway. We modelled the enzyme profiles by differential equations for each enzyme with including dilution due to cell growth. We considered a corresponding maximum slope due to enzyme synthesis rates by and the free protein synthesis capacity by where d max =0.01. Furthermore, we also integrated the influence of an optimal time varying growth by an additional differential equation for growth rate This can be interpreted as a dynamic adaption of growth rate due to environmental changes. We choose also a maximum adaption rate on the basis of a separate time domain, which is slower than the enzyme synthesis (here d μ, max =0.001). During pathway activation, the constraints in enzyme synthesis and growth adaption could cause high accumulations of metabolites, which are harmful to the cell [6] , [17] . We took this limitation into account by constraining total metabolite concentration with Ω =4 by The continuous optimization problem was transformed to a nonlinear programming problem by the quasi-sequential approach [40] . The quasi-sequential approach was extended to handle approximation errors in moving finite element strategies (called qMFE), with constraints on state and optimization variables [41] . In this work, we used qMFE also for problems with fixed final time to identify optimal time profiles independent of a predefined element placement. The optimal time courses of the enzymes e j ( t ) and growth rate profile μ ( t ) were computed numerically by using d j ( t ) and d μ ( t ) as decision variables. As we used a gradient-based approach [42] , to avoid local optima, we solved the problem 100 times with random initializations of the decision variables and choose only the results with the best objective value. Evaluation of optimization results To determine the position in the activation sequence ( Fig. 2 ), we sorted the activation times of enzymes in increasing order and determined for each enzyme its position in this ordered list. For the runs with randomized kinetic parameters, the abundances of enzymes (defined as the concentration after pathway activation) were normalized to an average of 1. We defined an enzyme as low abundant if its normalized abundance was <1 divided by 1.1 and as high abundant if it was >1.1. To determine the number of GpO, we grouped enzymes together in an operon if their activation time was not more than 1 time unit of the optimization apart (total simulation time was t f =1,000 time units). The activation time t active ,j of enzyme j was determined as the time when e j ( t active ,j )≥ d j, max , that is, when the concentration of enzyme j is above its maximal synthesis capacity for a time unit. For a given operonic organization resulting from the optimization, we determined the distribution of the positional coexpression bias as follows. First, we grouped enzymes according to the above definition into the sets ‘low abundant’ and ‘high abundant’. Then we determined for each co-occurrence of an enzyme within the high and low abundance sets with any other enzyme of the pathway in an operon the positional coexpression bias, that is, the distance in reaction steps. For instance, if the high abundance enzyme e 3 (that catalyses reaction 3) appears together with e 1 (that catalyses reaction 1) in an operon, this distance is −2 (relative to enzyme e3). For the low abundance enzyme e 2 , which occurs in the same operon like e 4 , this distance is +2. To construct the histogram in Fig. 3b , we counted the number of occurrences of each possible coexpression bias value and determined the frequency of each value for low and high abundance enzymes independently. We compared the distribution of positional coexpression values with the distribution we obtained from a purely random operonic organization. To this end, we determined the coexpression bias values for an operonic organization in which the identity of genes belonging to each operon has been randomly reassigned. To avoid bias due to a single randomization of operon structure, the distribution of coexpression bias from randomized operons summarizes the overall distribution obtained from 100 independent experiments with randomized operons. Genome annotation and codon adaptation indices The operon structure for the considered organisms was downloaded from MicrobesOnline [32] . General information on the number of protein-coding genes, sets of metabolic and non-metabolic genes, the copy-number of the rRNA operons and detailed information on the genome annotation of the organisms within MicroCyc [31] were obtained from the PathwayTools [43] files provided with the database. We could map information on operonic structure obtained from MicrobesOnline to 550 organisms from the MicroCyc collection. The codon adaptation indices contained within MicroCyc were provided by David Vallenet. Pathway structure and operonic organization To determine linear chains of reactions considered in our optimization, we used information on pathway structure provided from MetaCyc [44] . This database contains detailed layout information for each pathway that also allowed us to determine actual substrates and products within the pathway as well as cofactors. On the basis of the layout, we determined the reaction graph of each pathway (as displayed on the web interface of each pathway in the MetaCyc database) and defined the sequence of reactions within each pathway as the longest path between a metabolite that is not produced by any reaction of that pathway (pathway substrate) and a metabolite that is not produced by any other reaction of that pathway (pathway product). We determined the enzymes associated to each pathway as those that occurred in the longest path, as defined above. The number of GpO was computed as the number of enzymes associated to the pathway divided by the number of operons across which these enzymes are distributed. The average positional coexpression bias of low and high abundance enzymes of an organism was determined as follows. First, an enzyme was defined as low abundant if its codon adaptation index minus the average codon adaptation index of enzymes within a pathway was below −0.1 (codon adaptation indices range from 0 to 1). Enzymes were defined as high abundant if their codon adaptation index minus the average codon adaptation index of enzymes within the pathway was above 0.1. Results did not change significantly for small changes in these threshold values. For each organism, we determined the distribution of the positional coexpression bias values for high and low abundance enzymes for the actual and the randomized operonic structure, as in the analysis of the positional coexpression bias from the optimization results. We did not consider enzymes occurring in the same operon if they are associated to the same reaction to exclude bias due to enzymes that are coexpressed because they occur in a multi-enzyme complex. Subsequently, we determined the average positional coexpression bias for low and high abundance enzymes with actual and randomized operonic structure as the mean of the corresponding distributions. Statistical tests In the analyses of hypotheses about genomic features influencing operon sizes across different species, we considered the influence of the factors ‘ribosomal RNA copy-number’, ‘number of protein-coding genes’, ‘average codon adaptation index of proteins in the pathway’ (as a proxy for protein abundance) and ‘average non-metabolic operon size’. In all analyses, we determined the influence of each factor independently from the other factors on the size of operons in which enzymes for each particular pathway are organized. To this end, we computed partial correlations between each factor and operon sizes while controlling for the other investigated factors. Thus, when testing hypothesis 1 for a specific pathway (relationship between operon size and number of protein-coding genes), we computed the partial Spearman’s correlation between the operon size of genes of the specific pathway and the number of protein-coding genes while controlling for the number of rRNA operons, average protein abundance within the pathway and the average size of non-metabolic operons. Statistical evaluations were performed using R [45] . Partial correlations were computed using the R package ppcor. To test whether phylogenetic dependencies between species have an influence on our results, we repeated our analyses with reduced organism sets in which organisms belonging to particular clades were randomly removed. As described in Supplementary Note 6 , we could confirm that our results also apply to subsets of species from the MicroCyc collection. How to cite this article: Bartl, M. et al . Dynamic optimization identifies optimal programmes for pathway regulation in prokaryotes. Nat. Commun. 4:2243 doi: 10.1038/ncomms3243 (2013).